Ultrahigh-Q guided mode resonances in an All-dielectric metasurface High quality(Q) factor optical resonators are indispensable for many photonic devices. While very large Q-factors can be obtained theoretically in guided-mode settings, free-space implementations suffer from various limitations on the narrowest linewidth in real experiments. Here, we propose a simple strategy to enable ultrahigh-Q guided-mode resonances by introducing a patterned perturbation layer on top of a multilayer-waveguide system. We demonstrate that the associated Q-factors are inversely proportional to the perturbation squared while the resonant wavelength can be tuned through material or structural parameters. We experimentally demonstrate such high-Q resonances at telecom wavelengths by patterning a low-index layer on top of a 220 nm silicon on insulator substrate. The measurements show Q-factors up to 2.39 × 10 5 , comparable to the largest Q-factor obtained by topological engineering, while the resonant wavelength is tuned by varying the lattice constant of the top perturbation layer. Our results hold great promise for exciting applications like sensors and filters. High-Q photonic nano-resonators constitute a core element in high-performance optoelectronic and photonic devices in modern optical communications. While very large Q-factors have been obtained with micro-ring resonators and micro-disks via the optical fiber excitation through in-plane near-field coupling [1] , it is very challenging to achieve an ultrahigh Q-factor in experiments via free-space excitation. Resonant waveguide gratings and photonic crystal slab are viewed as an ideal platform to achieve high-Q guided-mode resonances (GMRs) [2] , [3] , [4] , which can be accessed in free space. They have been widely used in in filtering [5] , [6] , [7] , [8] , [9] , [10] , sensing [11] , [12] , [13] , and wavefront shaping [14] , [15] . Although the Q-factors of GMRs in theory can be very high, the largest Q-factor in experiments has been so far limited by fabrication imperfections (i.e., roughness, disorder and non-uniformity) causing increased radiation loss. The nanofabrication process usually involves dry-etching to define these nanostructures, introducing additional surface roughness [16] , imperfect vertical side walls [17] , and long-range non-uniformity [18] . 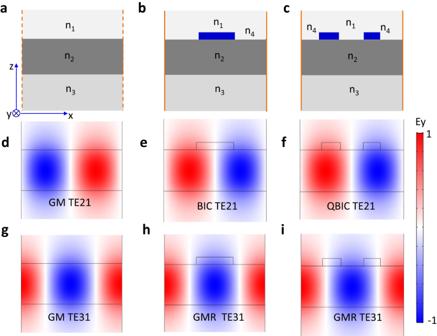Fig. 1: Designing strategy of high-Q GMRs. a–cSchematic drawing of a three-layer waveguide system (a), and meta-waveguide system with a top perturbation layer as simple grating (b) and compound grating (c) on the top.d,gare Ey distribution of GMs TE21and TE31.e,hare Ey distribution of symmetry protected BIC TE21and GMR TE31in the standard grating.f,iare Ey distribution of QBIC TE21and GMR TE31for the compound grating. To date, most of the reported Q-factors of GMRs in experiments fall in the range of from few hundreds to thousands, as summarized in Table 1 . High-Q resonances up to 2340 have been realized with plasmonic metasurfaces [19] by harnessing surface lattice resonances, but such plasmonic approaches are widely recognized to be limited by intrinsic material loss. Another candidate to achieve high-Q resonances is the all-dielectric metasurface exploiting electromagnetically induced transparency phenomena [20] . Table 1 Summary of measured Q-factor in the grating, photonic crystal slab, and metasurface Full size table Recently, bound states in the continuum (BICs) have introduced a viable alternative to realize ultrahigh-Q resonances in a free space setting [21] , [22] , [23] , [24] , [25] . The giant field enhancement typically associated with large-Q factors can benefit applications ranging from lasing [26] , [27] , [28] , [29] , [30] , sensing [31] , [32] , strong coupling [33] , [34] to enhanced nonlinear harmonic generations [35] , [36] , [37] , [38] . Most of the quasi-BICs(QBICs)-based high-Q modes reported so far are achieved by patterning the high-index semiconductor thin film as a single nanoparticle [39] , [40] , [41] or an array of nanoparticles on substrate [21] , [22] , [26] , [29] , [37] , [42] , [43] , [44] , [45] , [46] . Table 1 summarizes the measured Q-factor of QBIC modes based on all-dielectric metasurfaces. Typically, the Q-factors of QBICs are limited by scattering loss caused by unavoidable fabrication imperfections (i.e., roughness, disorder). Also, the presence of a substrate may also introduce the additional leaky channel due to out-of-plane asymmetry, further reducing the Q-factors of QBICs. Of course, ultrahigh-Q modes can still be constructed by carefully arranging the structure parameters. For example, topological BICs, arising from merging multiple BICs into a single one, are found to be less sensitive to fabrication imperfections [47] , [48] , [49] , [50] , [51] , [52] . However, achieving such a high Q-factor requires delicate engineering of the structure parameters and may not always be compatible with other design goals. Moreover, the substrate must be removed to satisfy the requirement for environmental symmetry. In addition, generalizing this achievement to visible wavelengths is an outstanding challenge that may prove difficult due to materials and fabrication constraints. To promote widespread adoption in practical applications, it is highly desirable to develop a universal yet simple design strategy to realize ultrahigh Q-resonances that minimize the impact of fabrication imperfections, mitigate the substrate effect, and do not need careful engineering based on complex topological concepts. In this work, we introduce a strategy to implement ultrahigh-Q guided-mode resonances in an all-dielectric metasurface without the need for topological engineering of the structure or introducing any symmetry breaking other than the discretization of translational symmetry. Instead of patterning the high-index layer to form a Mie resonator in a unit cell, we introduced an ultrathin photoresist layer as a perturbation layer on top of a multilayer-waveguide system so that guided modes are transformed into leaky modes that produce GMRs, which obviates the need for dry-etching. High Q-factors of GMRs can be easily realized as they are inversely proportional to the perturbation parameter squared (Q ∝ α −2 ). The perturbation can be reduced to a very small value because the fabrication of such a device only involves spin-coating of resist and developing, enabling minimal perturbation by removing the roughness and disorder of the sample. The validity of such a design methodology is confirmed by patterning a low-index photoresist thin film on a standard silicon on insulator (SOI) sample that serves as a simple waveguide system. The experimental results show that the Q-factor was as high as 2.39 × 10 5 , comparable to the maximum Q-factor of topological BICs. In addition, the resonant wavelength was easily tuned by changing the period of the meta-waveguide system. This design strategy is robust and powerful in obtaining ultrahigh-Q resonances at arbitrary operating wavelengths because it can be generalized to any other waveguide system made of any different high refractive index ( n = 2 ∼ 5) as the core layer. Our results may find great potential in applications requiring very sharp spectral features, such as sensing and filtering. Guided modes in a multilayer-waveguide system We start by investigating the leaky modes of a multilayer waveguide structure, consisting of a high refractive index n 2 layer with finite thickness sandwiched between two semi-infinite layers with low refractive index being n 1 and n 3 , respectively. Without loss of generality, we assume that the electric field component is perpendicular to the plane of structure, which is E//y. Such an open system supports a series of Fabry-Perot resonant modes with low-Q factors (See Section 1 of supplementary materials and Fig. S 1 ). If we apply a virtual periodic boundary condition with arbitrary periods, in addition to the low-Q leaky modes, such a simple geometry can also support guided modes (GMs) with an infinite Q-factor. Note that there are two ways of defining a periodic structure: a 1D grating or a 2D metasurface, as shown in Fig. 1a and Fig. S 2 . The band diagram for TE (E//y) and TM (H//y) modes can be obtained by folding the waveguide dispersion of GMs into the first Brillouin zone. The dispersion relationship of GMs has been derived in the text book [53] and can be expressed as follows 
    TE:tan(β_2t)=β_2(β_1+β_3)/β_2^2-β_1β_3
 (1) 
    TM:tan(β_2t)=n_2^2β_2(β_1+n_3^2β_3)/n_3^2β_2^2-n_2^2β_1β_3
 (2) Where \({\beta }_{1}=\sqrt{{k}^{2}-{{n}_{1}^{2}k}_{0}^{2}}\) , \({\beta }_{2}=\sqrt{{{n}_{2}^{2}k}_{0}^{2}-{k}^{2}}\) , \({\beta }_{3}=\sqrt{{k}^{2}-{{n}_{3}^{2}k}_{0}^{2}}\) , \(k\) is the propagating constants of guided mode, \({k}_{0}=\omega /c\) , ω is the angular frequency and c is the speed of light in the vacuum. Fig. 1: Designing strategy of high-Q GMRs. a – c Schematic drawing of a three-layer waveguide system ( a ), and meta-waveguide system with a top perturbation layer as simple grating ( b ) and compound grating ( c ) on the top. d , g are Ey distribution of GMs TE 21 and TE 31 . e , h are Ey distribution of symmetry protected BIC TE 21 and GMR TE 31 in the standard grating. f , i are Ey distribution of QBIC TE 21 and GMR TE 31 for the compound grating. Full size image It is necessary to mention that there is a cut-off frequency for different guided modes. Ω_cj=c/t√(n_2^2-n_3^2)(tan^-1[s√(n_3^2-n_1^2/n_2^2-n_3^2)]+jπ)(j=0,1,2… )
 (3) Where s = 1 for TE and \({s=n}_{2}^{2}\) , c is the speed of light in the vacuum. More detailed discussions on band structure calculation are given in section 2 of supplementary materials and Fig. S 3 . Guided mode resonances and BICs Here, we mainly focus on the GMs at Γ-point in the first Brillouin zone in momentum space. Alternatively, the eigenfrequencies of these GMs can be calculated quickly with the commercial software COMSOL Multiphysics. For the 1D grating system, these GMs are designated as TE ml (TM ml ) [54] , [55] , where m and l are the numbers of antinodes of the electric (magnetic) field in the x and z directions, respectively. Fig. 1b, c shows two typical examples of GMs: modes TE 21 and TE 31 . These GMs can be transformed into GMRs by introducing an ultrathin low-index metasurface on top of the high-index layer. For example, when the top perturbation layer is patterned as a grating, GMs TE 21 and TE 31 are converted into symmetry-protected BIC mode TE 21 and GMR TE 31 with a finite Q-factor, respectively. If the mirror symmetry of the top periodic structure is broken with respect to the z-axis, BIC mode TE 21 is reduced to QBIC. Note that GMs like TE 21 and TE 31 at the Γ point share a similar feature with symmetry protected BICs. When the periodic perturbation is introduced in the multilayer waveguide system, such GMs with infinite Q-factors are successfully converted into either a BIC mode with an infinite Q-factor or a GMR with a finite Q-factor depending on the mode parity. If the perturbation approaches zero, the radiative decay rates of GMRs are reduced to zero. Rigorous derivation shows that Q values are inversely proportional to β 2 (see section 3 of supplementary materials), where β is the perturbation parameter of the system. This is similar to the symmetry-protected BICs with Q ∝ α −2 (where α is the asymmetry parameter of unit cell). The GMs for the TM case are shown in Fig. S 4 . The following sections demonstrate that GMs provide much freedom and flexibility to design ultrahigh Q-factor resonance with a subwavelength meta-waveguide system at an arbitrary operating wavelength. For simplicity, we use a three-layer structure air/Si/SiO 2 to design a high-Q resonance at λ 0 = 1550 nm. Without loss of generality, the thickness of the middle layer Si is chosen as 220 nm. The refractive index of Si and SiO 2 are set as 3.47 and 1.46, respectively. The dispersion relationship of GMs in such a three-layer system can be obtained from Eq. ( 1 ) and is shown in Fig. 2 . To support a GM at λ 0 = 1550 nm (dashed black line in Fig. 2 ), the propagation constants should be \(\,k=5.6515*{{{{{\rm{\pi }}}}}}/{\lambda }_{0}\) . Then, the virtual period can be obtained as p = 548 nm by applying \(k=2{{{{{\rm{\pi }}}}}}/p\) . In principle, the resonant wavelength can be tuned to any other value by varying the period, which is discussed in the later section. Fig. 2: Dispersion relationship of GMs in a multilayer system (air/220 nm Si/SiO 2 ). Solid blue and red lines corresponds to GMs TE0 and TE1, respectively. The dashed black line indicates the GM wavelength at 1550 nm. Full size image By introducing a top perturbation layer that is patterned as either a grating or a metasurface, the GM evolves into a BIC or GMR depending on the structure’s geometry and the mode’s parity. Their band structures are plotted in Figs. S 5 , 6 . Here, it is worth noting that the refractive index of grating or metasurface can be of any value as long as the top layer serves as a perturbation layer. As an example, the refractive index of the top layer is set as 1.46, matching the index of SiO 2 . We first consider a simple grating structure shown in Fig. 3a and study the effect of width and thickness on the Q-factor of GMR. From Fig. 3b , it can be found that the Q-factor of the GMR TE 31 is proportional to t −2 when the width of the grating is fixed as 200 nm. Excellent agreement can be found between the calculated Q-factor (solid red line) and fitted Q-factor (dashed blue line) by applying the fitting equation Q=Ct −2 (C is the fitted constant). This is similar to the observation in symmetry-protected BICs, where Q ∝ α −2 (where α is the asymmetry parameter). Such a relationship is well explained by perturbation theory [56] (see section 3 in supplementary materials). This is also confirmed by the reflection spectrum mapping as the thickness increases from 0 to 300 nm (See Fig. S 7 ). Fig. 3: High-Q GMRs. a Schematic drawing of a meta-waveguide system made of an ultrathin SiO 2 grating on top of 220 nm-Si on SiO 2 substrate. b The Q-factor of GMR mode TE 31 vs thickness of top perturbation layer. Solid and dashed lines refer to the numerically calculated Q-factor and fitting Q-factor. The structure parameters are p = 548 nm and w = 200 nm. c The Q-factor of GMR mode TE 31 vs grating’s width. Solid and dashed lines show the numerically calculated Q-factor and fitting Q-factor. The structure parameters are p = 548 nm and t = 40 nm. d Schematic drawing of a meta-waveguide system made of an ultrathin SiO 2 compound grating on top of 220 nm-Si on SiO 2 substrate. e The Q-factor of QBIC TE 21 (solid red) and GMR TE 31 (solid blue) vs thickness of top perturbation layer. Dashed lines are fitting Q-factor. The structure parameters are p = 548 nm, w = 110 nm, d = 90 nm, g = 120 nm, xc = 10 nm. f The Q-factor of BIC TE 21 (solid red) and GMR TE 31 (solid blue) vs gap center xc. The structure parameters are p = 548 nm, w + d = 200 nm, g = 120 nm. Dashed lines are fitting Q-factors. g Schematic drawing of a meta-waveguide system made of an ultrathin SiO 2 metasurface on top of 220 nm-Si on SiO 2 substrate. h The Q-factor of GMR mode TE 311 vs the thickness of top perturbation layer. Solid and dashed lines show the numerically calculated Q-factor and fitting Q-factor. The structure parameters are p = 548 nm, w = 200 nm. i The Q-factor of BIC TE 211 (solid red) and GMR TE 311 (solid blue) vs top layer thickness. Dashed lines are fitting Q-factor. The structure parameters are p = 548 nm, w + d = 200 nm, g = 120 nm. Full size image Similarly, the Q-factor shows a linear dependence on w −2 or (d-w) −2 for a given thickness, as confirmed in Fig. 3c . Thus, it can be safely concluded that the effective perturbation area or volume plays the dominant role in governing the Q-factors of GMRs. Moreover, the resonant wavelength remains almost the same with the changing thickness or width because of the low-index nature of the top perturbation layer (See Figs. S 7 , 8 ). As described in Fig. 1 , except for the GMR TE 31 , such a grating also supports a symmetry-protected BIC mode TE 21 due to structural symmetry. Further breaking the symmetry can induce the transition from BIC to QBIC. For instance, by introducing an asymmetric air slit inside the rectangular nanowire, BIC mode TE 21 is successfully converted into the QBIC. Fig. 3b shows the Q-factor of QBIC TE 21 as a function of thickness. The case of TE 31 is also plotted as a reference to make a comparison in Fig. 3d–f . Similar to the case of TE 31 shown in Fig. 3b , the Q-factor of QBIC TE 21 is proportional to t −2 when an asymmetric slit is introduced with g = 120 nm and xc = 10 nm. The left and right nanowires’ widths are 110 nm and 90 nm, respectively. Besides, we find that the Q-factor of QBIC mode TE 21 is more than one order of magnitude higher than that of mode TE 31 . This is understandable because the perturbation required for symmetry-breaking is much smaller for QBIC TE 21 compared to GMR TE 31 . Such a general conclusion also can be applied to the 3D metasurface. When the cuboid unit cell of the top perturbation layer is arranged as a square lattice, such a metasurface supports degenerate symmetry-protected BICs (TE 211 and TE 121 ) and GMRs (TE 311 and TE 131 ). The degeneracy could be easily lifted by choosing the different lattice constants along the x and y-axis (See Fig. S 9 ). Further introducing in-plane broken symmetry leads to the transition from BICs into QBICs for the TE 211 mode. Fig. 3g–i shows the Q-factor of GMR TE 311 and QBIC TE 211 versus the thickness of top layer. Additionally, it is not surprising that Q-factor follows a similar trend as 1D grating, Q ∝ t −2 . Moreover, such a 2D metasurface supports BICs or GMRs for TM cases (See Fig. S 10 ). Here, it is necessary to point out that the top layer can also be patterned as a rectangular lattice with any other shape such as photonic crystal slab because it just functions as a weak perturbation layer. Guided mode resonances engineering Note that many GMs can be easily constructed with such a simple meta-waveguide system. We again consider the 1D grating structure shown in Fig. 1a with material parameters and geometry parameters given in Fig. 3a . Except for TE 21 and TE 31 mode, such a three-layer structure supports other high-order GMs. Fig. 4a shows the field distributions of six GMs: TE 21 and TE 31 , TE 22 and TE 32 , TE 41 and TE 51 . Their resonant wavelengths are presented in Fig. 4b . Note that all of these modes are dominated by the zero-order diffraction. Of course, even higher-order GMs like TE 42 and TE 52 can be found. However, their Q-factor may decrease significantly due to the enhanced radiation from unwanted diffraction after the perturbation is introduced. Also, GMs may be designed at any pre-defined wavelength with different structure parameters and material parameters. For example, if the thickness of the Si layer is set as 220 nm or 340 nm, we can always tune the virtual period so that the resonant wavelengths of GM TE 21 or TE 31 could cover a broadband wavelength range from 1000 nm to 1800 nm, as displayed in Fig. 4c . Fig. 4: Designing GMs at arbitrary wavelengths. a Eigenfield distributions Ey of six GMs in the 220 nm-Si on SiO 2 substrate with virtual period p = 548 nm. b Resonant wavelengths of six GMs. The dashed line indicates the first-order diffraction wavelength. c Resonant wavelength engineering through the virtual period for GMs TE 21 and TE 31 . The dashed lines indicate the resonant wavelength 1550 nm (black) and 1350 nm (magenta). d Resonant wavelength engineering through the thickness of Si layer for GMs TE 21 and TE 31 . The dashed lines indicate the resonant wavelength 1550 nm (black) and 1350 nm (magenta). e Virtual period of three-layer waveguide as a function of refractive index of middle layer for GMs TE 21 and TE 31 . Here, the resonant wavelengths of two GMs are fixed as 1550 nm. f Q-factors of GMR TE 31 vs the thickness of top perturbation layer for the meta-waveguide system with varied refractive index of middle layer. Full size image Similarly, from Fig. 4d , we found that the resonant wavelength can be tuned by varying the thickness of Si layer while the period is fixed as 450 nm (or 550 nm). One can also engineer the GM’s wavelength by choosing materials with different refractive indices. For example, to design a GM at 1550 nm, the period should be varied from 1000 nm to 460 nm when the refractive index n 2 increases from 2 to 4. The corresponding result is shown in Fig. 4e . To verify the robustness of such a design strategy in realizing ultrahigh-Q resonances, we calculate the Q-factor of GMR TE 31 in a grating system for the middle layer with various refractive index n 2 . Indeed, all of the Q-factors decrease significantly with the increasing thickness of the top grating layer, as illustrated in Fig. 4f . Nevertheless, it is interesting that the Q-factor for high-index n 2 = 3.5 is almost one order higher than the low-index n 2 = 2.0. This can be intuitively understood by the reduced index contrast between the substrate (or superstrate) and the sandwiched high-index layer, which leads to more energy radiation into the substrate (or superstrate) instead of confining inside the high-index layer. The robustness of such a design strategy could enable us to design ultrahigh-Q GMRs at ultraviolet and visible wavelength ranges by choosing appropriate core layers with high-index, including Si 3 N 4 , GaN, TiO 2 . In the supplementary materials, we demonstrate two examples of designing high-Q resonators in the visible wavelength by using GaN and Si 3 N 4 as core layer, as shown in Figs. S 11 , 12 . Experimental demonstrations of high-Q GMRs After gaining a solid understanding of designing ultrahigh-Q resonances from GMs, we move to the experimental demonstration of such a high-Q resonance. Fig. 5 shows the experimental setup of a custom-made crossed-polarization measurement system. Crossed polarization measurement has been widely used to measure the high-Q resonances [50] , [57] . We fabricate a series of photonic crystal slabs made of 330 nm thick photoresist (ZEP520) on an SOI substrate (220 nm-Si/2 µm-SiO 2 /Si) using electron-beam lithography followed by developing process. Here, the photo-resist layer instead of the SiO 2 layer is patterned as a perturbation layer. On the one hand, the photoresist has a low refractive index of around 1.4. On the other hand, no other post-processing (i.e., dry etching) is applied to the other layers so that higher sample quality is guaranteed. Fig. 5: Schematic illustration of experimental setup. Light red and light blue lines indicate the incident light and direct reflection from the sample, respectively. 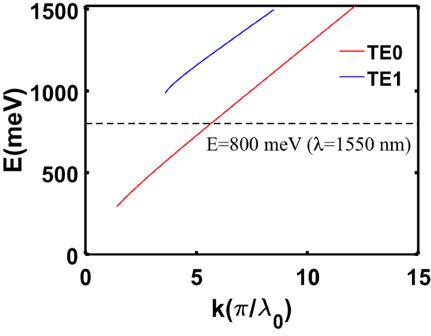Fig. 2: Dispersion relationship of GMs in a multilayer system (air/220 nm Si/SiO2). Solid blue and red lines corresponds to GMs TE0 and TE1, respectively. The dashed black line indicates the GM wavelength at 1550 nm. L means lens and BS means beam splitter. Full size image Fig. 6a shows the schematic drawing of the whole device, and Fig. 6b shows the scanning electron microscopy image of one typical fabricated sample. The lattice constants along the x- and y-axis are identical in this device. We first investigate the effect of hole size on the Q-factor by fixing the lattice constant as 545 nm but varying the hole radius. Eigenmode calculations indicate that such a structure can support degenerate GMRs TE 311 and TE 131 at around 1550 nm. It also supports symmetry protected BICs TE 211 and TE 121 . However, they cannot be excited at normal incidence unless the in-plane mirror symmetry is broken with respect to the y-z plane. Fig. 6: Experimental demonstration of high-Q resonances based on GMs. a Schematic drawing of a 3D meta-waveguide system. The top perturbation is patterned as photonic crystal slab with air hole. b SEM image of a fabricated meta-waveguide system. The scale bar in white is 200 nm. c Eigenfield distribution for GMR TE 311 . d Measured reflection spectra for four fabricated samples with fixed period 545 nm but varied hole radius from 72 nm to 105 nm. e Fano-fitting for reflection spectrum for hole radius R = 72 nm. f Retrieved Q-factors vs radius for mode TE 311 , dash line is the simulated Q-factor. g Measured reflection spectra for a meta-waveguide system when periods change from 535 nm to 555 nm. h Comparison between calculated and measured resonant wavelength. i Retrieved Q-factors vs period. a.u in the figure the abbreviation of arbitrary units. Full size image The relevant results are put in Fig. 6d–f . It can be observed from Fig. 6d that shrinking the size of the hole on the top perturbation layer leads to the narrowing of resonance linewidth and slight redshift of resonance. We retrieved the Q-factors and resonant wavelengths of these high-Q resonances by fitting them to a Fano-profile. Fig. 4e shows one example of Fano fitting for R = 72 nm. The measured Q-factor for structures with different hole sizes is presented in Fig. 6f , where the highest Q-factor is up to 2.39 × 10 5 at R = 72 nm. Such a high Q-factor is comparable to the record-high Q-factors in a topological metasurface [50] . Nevertheless, our approach involves only patterning the top resist layer without the need for carefully engineering the topological features. Also, the calculated Q-factor is plotted as a reference and is found to show an excellent agreement with the experiment measurement. 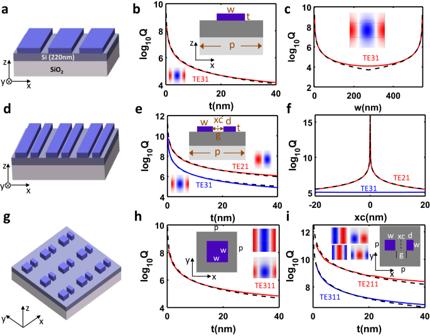Fig. 3: High-Q GMRs. aSchematic drawing of a meta-waveguide system made of an ultrathin SiO2grating on top of 220 nm-Si on SiO2substrate.bThe Q-factor of GMR mode TE31vs thickness of top perturbation layer. Solid and dashed lines refer to the numerically calculated Q-factor and fitting Q-factor. The structure parameters arep= 548 nm andw= 200 nm.cThe Q-factor of GMR mode TE31vs grating’s width. Solid and dashed lines show the numerically calculated Q-factor and fitting Q-factor. The structure parameters arep= 548 nm andt= 40 nm.dSchematic drawing of a meta-waveguide system made of an ultrathin SiO2compound grating on top of 220 nm-Si on SiO2substrate.eThe Q-factor of QBIC TE21(solid red) and GMR TE31(solid blue) vs thickness of top perturbation layer. Dashed lines are fitting Q-factor. The structure parameters arep= 548 nm,w= 110 nm,d= 90 nm,g= 120 nm, xc = 10 nm.fThe Q-factor of BIC TE21(solid red) and GMR TE31(solid blue) vs gap center xc. The structure parameters arep= 548 nm,w+ d = 200 nm,g= 120 nm. Dashed lines are fitting Q-factors.gSchematic drawing of a meta-waveguide system made of an ultrathin SiO2metasurface on top of 220 nm-Si on SiO2substrate.hThe Q-factor of GMR mode TE311vs the thickness of top perturbation layer. Solid and dashed lines show the numerically calculated Q-factor and fitting Q-factor. The structure parameters arep= 548 nm,w= 200 nm.iThe Q-factor of BIC TE211(solid red) and GMR TE311(solid blue) vs top layer thickness. Dashed lines are fitting Q-factor. The structure parameters arep= 548 nm,w+ d = 200 nm,g= 120 nm. In fact, we also fabricate the sample with an even smaller radius R = 35 nm. However, it becomes very challenging to get an even higher Q-factor in experiment because the peak cannot be distinguished from the noise or background. Further optimization of the measurement system is needed. Such an ultrahigh-Q factor can be attributed to two factors: small hole radius and shallow hole with partial unetched resist film underneath. After taking both factors into account, the calculated Q is an order of million for such a size (See Fig. 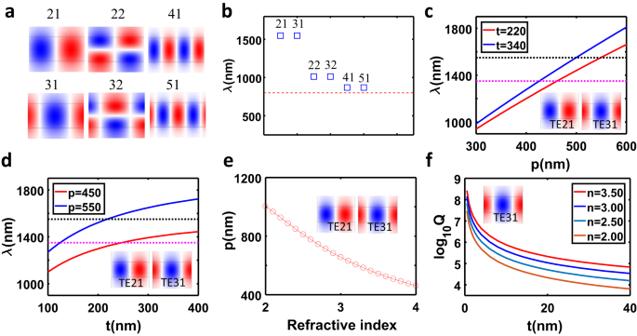Fig. 4: Designing GMs at arbitrary wavelengths. aEigenfield distributions Ey of six GMs in the 220 nm-Si on SiO2substrate with virtual periodp= 548 nm.bResonant wavelengths of six GMs. The dashed line indicates the first-order diffraction wavelength.cResonant wavelength engineering through the virtual period for GMs TE21and TE31. The dashed lines indicate the resonant wavelength 1550 nm (black) and 1350 nm (magenta).dResonant wavelength engineering through the thickness of Si layer for GMs TE21and TE31. The dashed lines indicate the resonant wavelength 1550 nm (black) and 1350 nm (magenta).eVirtual period of three-layer waveguide as a function of refractive index of middle layer for GMs TE21and TE31. Here, the resonant wavelengths of two GMs are fixed as 1550 nm.fQ-factors of GMR TE31vs the thickness of top perturbation layer for the meta-waveguide system with varied refractive index of middle layer. S 13 ). Finally, to demonstrate the tunability of resonant wavelength, we fabricate five samples with the period varying from 535 nm to 555 nm while their hole radii are fixed as 80 nm. The scattering spectra are plotted in Fig. 6g . Indeed, the resonant peaks show a linear dependence on the period (Fig. 6h ), matching very well to the theoretical calculation. In addition, all of the measured Q-factor are ranged between 1.0 × 10 5 and 2.0 × 10 5 (Fig. 6i ). Note that TE 311 and TE 131 are degenerate for the identical lattice constants along the x and y-axis. This degeneracy can be lifted by employing a rectangular lattice with different p x and p y . Thus, high-Q resonance could be implemented at a different wavelength by switching the polarization (See Fig. S 14 ). In other words, even a single structure can support two high-Q modes at different wavelengths for x and y-polarization. An even higher-Q factor can be obtained by exciting QBICs via breaking the unit-cell’s mirror symmetry, as demonstrated in Fig. 3i . In addition to reducing the hole size, such an ultrahigh-Q mode may be enabled by using an ultrathin material as a perturbation layer. The recently developed two-dimensional (2D) materials, especially 2D transition metal dichalcogenides (TMDCs) [58] , [59] and hexagonal boron nitride (hBN) [60] , are ideal candidates for realizing atomically thin film below 10 nm. Moreover, such a 2D TMDC multilayer with thickness below 10 nm can be easily patterned by induced coupled plasma (ICP) etching. Although the refractive index of TMDC is a bit high ( n = 3 ∼ 4.5 in the near-infrared), their atomically thin nature makes them an excellent candidate as a perturbation layer. We expect a high-quality thin film like TMDCs and hBN multilayers, and mature fabrication process could help to realize an ultrahigh-Q factor larger than 10 6 or even more. Note: The results presented in this work are in bold. EIT-electromagnetic induced transparency; SLR- surface lattice resonance; GMR-guided mode resonance; BIC-bound state in the continuum; NP-nanoparticle; PCS-photonic crystal slab; SOI-silicon on insulator. In summary, we theoretically proposed and experimentally demonstrated high-Q guided resonances in a meta-waveguide system. The designing strategy builds upon adding a perturbation layer (i.e., photoresist) on top of a conventional waveguide system, which converts GMs into the BICs or GMRs. The Q-factors of GMRs strongly depend on the perturbation of a meta-waveguide system, suggesting a broadly adaptable way of realizing ultrahigh-Q resonances without resorting to topological concept, as demonstrated in the recent literature [46]. The ultrahigh Q-factor of GMRs can be realized because the fabrication of proposed structure only involves resist-coating and developing, but no deep etching process, successfully eliminating the common source of roughness and disorder of the sample and enabling a controlled tiny perturbation in realistic devices. We experimentally demonstrated the feasibility of this design strategy in achieving high-Q resonances at around 1.55 µm by fabricating a thin photoresist layer photonic crystal slab on top of 220 nm Si/2 μm SiO 2 /Si (standard SOI sample). The measured Q-factor reaches up to 2.39 × 10 5 , comparable to the value of merging BICs by topological charge engineering. Also, the resonant wavelength can be tuned by varying the lattice constant of the top resist layer. Furthermore, by choosing different lattice constants along the x- and y-axis, we realized polarization-dependent GMRs. Our findings open a new avenue to design optoelectronic and photonic devices in which ultra-sharp spectral features may improve their performance, such as biosensors and filters. 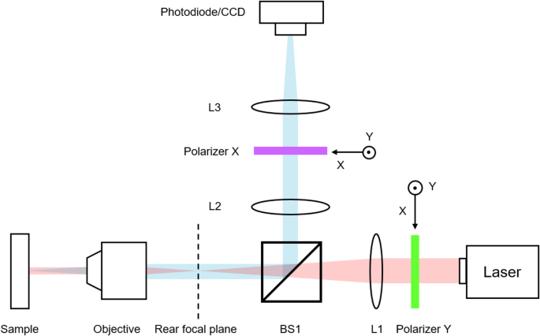Fig. 5: Schematic illustration of experimental setup. Light red and light blue lines indicate the incident light and direct reflection from the sample, respectively. L means lens and BS means beam splitter. 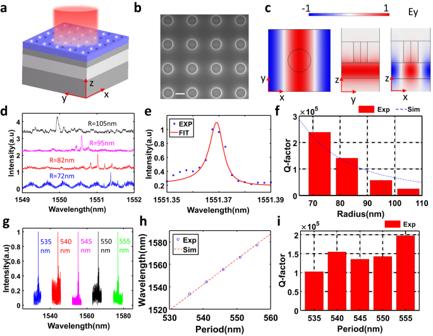Fig. 6: Experimental demonstration of high-Q resonances based on GMs. aSchematic drawing of a 3D meta-waveguide system. The top perturbation is patterned as photonic crystal slab with air hole.bSEM image of a fabricated meta-waveguide system. The scale bar in white is 200 nm.cEigenfield distribution for GMR TE311.dMeasured reflection spectra for four fabricated samples with fixed period 545 nm but varied hole radius from 72 nm to 105 nm.eFano-fitting for reflection spectrum for hole radiusR= 72 nm.fRetrieved Q-factors vs radius for mode TE311, dash line is the simulated Q-factor.gMeasured reflection spectra for a meta-waveguide system when periods change from 535 nm to 555 nm.hComparison between calculated and measured resonant wavelength.iRetrieved Q-factors vs period. a.u in the figure the abbreviation of arbitrary units. Numerical simulation The eigenmodes of meta-waveguide are calculated by commercial software Comsol Multiphysics based on finite-element-method (FEM). The reflection and transmission spectra of meta-structures are calculated by rigorous-coupled wave analysis (RCWA). Fabrication Our devices were fabricated on a silicon-on-insulator (SOI) wafer with a 220 nm silicon layer and 2 μm-thick buried layer. The SOI was firstly coated with the 330 nm-thick resist layer (ZEP520). Then, the device patterns were defined on the resist by electron-beam lithography. After that, the devices were carefully developed and fixed by dimethyl benzene and iso-Propyl alcohol, respectively. Optical Characterization The incident light source was a tunable telecommunication laser (santec TSL-550), the wavelength of which could be tuned from 1480 nm to 1630 nm. Light first passed through the polarizer, lens and beam splitter, and then focused on the rear focal plane of the objective lens (10X), to make sure the incident light on the sample was close to normal incidence. The reflected signal was collected by a photodiode (PDA10DT-EC), which could be switched to a CCD to locate the sample. A lock-in amplifier with the help of chopper (SR540) was connected to the photodiode to pick out the signal from the background noise. A pair of orthogonal polarizers were placed at the front and the middle part of the light path, to introduce crossed-polarization which could efficiently decrease the impact from background reflection and promote the relative intensity of the signal.